A Krüppel-like factor downstream of the E3 ligase WWP-1 mediates dietary-restriction-induced longevity inCaenorhabditis elegans The HECT ubiquitin E3 ligase WWP-1 is a positive regulator of lifespan in response to dietary restriction (DR) in Caenorhabditis elegans . However, substrates of WWP-1 for ubiquitylation in the DR pathway have not yet been identified. Here we identify the C. elegans Krüppel-like factor, KLF-1, as an essential and specific regulator of DR-induced longevity and a substrate for ubiquitylation by WWP-1. Knockdown of klf-1 suppresses the extended lifespan of both DR animals and wwp-1 -overexpressing animals, indicating that KLF-1 functions within the same pathway as WWP-1. In addition, overexpression of klf-1 in the intestine is sufficient to extend the lifespan of WT animals on an ad libitum diet, and requires wwp-1 or pha-4 /FoxA. We demonstrate that WWP-1 directly interacts with KLF-1 and mediates multiple monoubiquitylation of KLF-1 in vitro and in cellulo. Our data support a model in which modulation of KLF-1 by WWP-1 regulates diet-restriction-induced longevity. The Krüppel-like factor (KLF) family of gene regulatory proteins are transcription factors implicated in many biological processes that include proliferation, differentiation, growth, development, survival and responses to external stress [1] . The characteristic feature of KLF family members is the presence of three Krüppel-like zinc fingers at the carboxy (C)-terminus, which bind to CACCC elements and GC-rich regions of DNA, to mediate activation and/or repression of transcription. In addition, KLF proteins have nuclear localization sequences, which occur immediately adjacent to, or within, the zinc-finger motifs. The amino (N)-terminal regions of KLF proteins are much more variable, allowing the interaction with different coactivators, corepressors and modifiers, resulting in functional diversity and specificity. KLF proteins are present in species ranging from Caenorhabditis elegans to humans, with humans having at least 17 members. Three KLFs are predicted from the C. elegans genome: klf-1 (F56F11.3), klf-2 (F53F8.1) and klf-3 (F54H5.4). All three KLFs share the highest sequence identity with members of mammalian KLFs in the C-terminal C 2 H 2 domains but little homology in their N-terminal regions. Roles for klf-1 in fat regulation, germline cell death and phagocytosis have been described [2] , [3] . klf-3 (also known as mua-1 ) has been implicated in fat metabolism and cell matrix attachment [4] , [5] , [6] , [7] . KLF members participate in regulation of gene transcription through the interaction with intracellular signalling molecules and transcriptional cofactors. In addition, coregulatory proteins modify KLF family members via acetylation, phosphorylation, ubiquitylation and sumoylation to refine their transcriptional activity [1] . These post-translational modifications are thought, at least in part, to affect KLF family interactions with transcriptional cofactors, thus mediating the differential biological effects of KLFs. The mammalian family of WW domain-containing HECT E3 ligases has been shown to promote conjugation of ubiquitin to several KLF family members resulting in different protein fates. Mammalian WWP1 has been shown to mediate ubiquitylation of both KLF2 and KLF5, targeting these proteins for degradation [8] , [9] , [10] . Itch promotes monoubiquitylation of TIEG1/KLF10 and enhances its transcriptional activation of the Foxp3 promoter and Foxp3 expression [11] . Itch has also been shown to target phosphorylated TIEG1/KLF10 for K27-linked polyubiquitylation and prevent its nuclear translocation [12] . We previously identified the C. elegans WWP-1 E3 ligase and its associated E2 ubiquitin-conjugating enzyme, UBC-18, as positive regulators of lifespan in response to DR [13] . WWP1 is an E3 ubiquitin ligase orthologous to human WWP1, WWP2 and Itch. In addition to their C-terminal catalytic HECT domain, these ligases have an N-terminal Ca 2+ /lipid-binding C2 domain and four WW domains, modular protein-interaction domains that recognize short proline motifs in target proteins. While the ubiquitin ligase activity of WWP-1 is essential for DR-induced longevity, a substrate for WWP-1 to modulate this response is still unknown. Here we demonstrate that a C. elegans KLF, KLF-1, is a substrate for ubiquitylation by WWP-1. Like wwp-1 , klf-1 is essential and specific for the longevity response to decreased nutrient intake. In addition, genetic analysis reveals that klf-1 and wwp-1 function together within the intestine to modulate longevity in response to DR. klf-1 is required for the extension of lifespan by DR Loss of wwp-1 function suppresses the extended longevity of eat-2 mutant animals, a genetic model for DR, and other forms of diet restriction [13] . To identify potential substrates of WWP-1 that regulate DR-induced longevity, we performed a targeted RNAi screen by selecting worm orthologues of known ubiquitylated substrates of mammalian WWP-1 family members (WWP-1, WWP2 and Itch). None of the 12 genes we analysed were able to extend lifespan in wild-type (N2) worms when knocked down ( Fig. 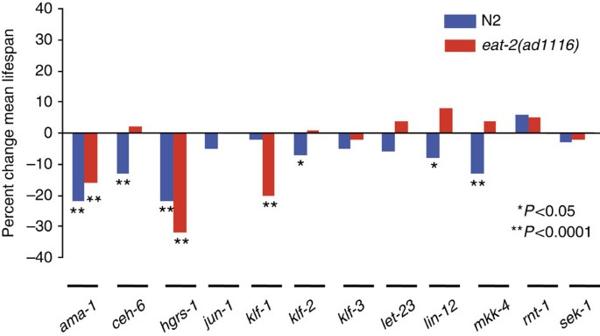Figure 1: Targeted RNAi screen to identify WWP-1 substrates involved in lifespan regulation. Percent change in mean lifespan in N2 worms (blue) oreat-2(ad1116)worms (red) treated with RNAi to the indicated genes only during adulthood compared with empty vector. Mean percent change of 1–4 independent experiments is shown. *P<0.05, **P<0.0001 (compared with same strain worms grown on HT115 bacteria harbouring the RNAi plasmid vector; Mantel–Cox log-rank test). Lifespan values are given inSupplementary Table 1. 1 and Supplementary Table 1 ). However, we found that loss of one gene, klf-1 , completely suppressed the extended longevity of eat-2 mutant animals but did not affect N2 lifespan ( Fig. 2a and b , Supplementary Fig. 1a and b and Supplementary Tables 2 and 3 ). This suppression appears to be exerted during adulthood, as we still observed this effect when we initiated RNAi at day 1 of adulthood ( Fig. 2a ). Previous studies have found that klf-1 knockdown affects egg-laying behaviour [3] . To rule out the possibility that the reduced lifespan noted on loss of klf-1 is due to premature death caused by egg-laying defects, we repeated the lifespans in a temperature-sensitive sterile background ( eat-2(ad1116); CF512: fer-15(b26);fem-1(hc17) ) and still observed complete suppression of lifespan with loss of klf-1 ( Supplementary Fig. 1c and Supplementary Table 3 ). 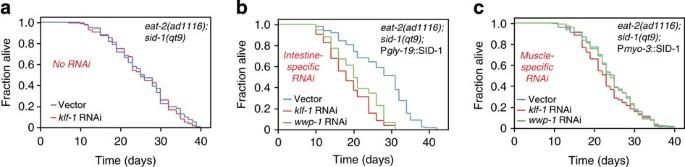Figure 3: The intestine is a major site of action ofwwp-1andklf-1to regulate the dietary restriction response. (a) Lifespan analysis ofeat-2(ad1116);sid-1(qt9)mutant worms fed bacteria expressing dsRNA toklf-1or control vector. (b,c) Lifespan analysis ofeat-2(ad1116);sid-1(qt9)worms with restored SID-1 expression in the intestines (b) or muscle tissues (c). Worms were fed bacteria expressing dsRNA toklf-1,wwp-1or control vector. The suppression of DR-extended lifespan by klf-1 depletion is unlikely to be due to increased food intake because no difference in pharyngeal pumping rates with knockdown of klf-1 in N2 or eat-2(ad1116) worms was observed ( Supplementary Table 4 ). 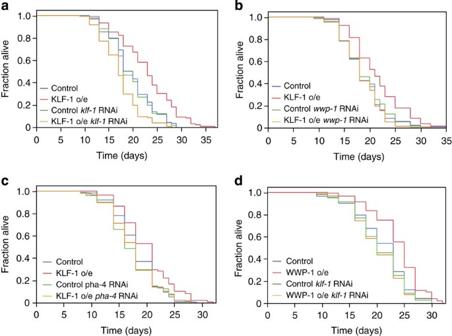Figure 4:wwp-1andklf-1function together to regulate diet-restriction-induced longevity. (a–c) Lifespan analysis of worms overexpressing KLF-1 in the intestine (KLF-1 o/e) or control worms fed bacteria expressingklf-1(a),wwp-1(b) orpha-4(c) dsRNA from hatching (L1) or control vector. (d) Lifespan analysis of WWP-1-overexpressing worms (WWP-1 o/e) or control worms fed bacteria expressingklf-1dsRNA from hatching (L1) or control vector. Figure 1: Targeted RNAi screen to identify WWP-1 substrates involved in lifespan regulation. Percent change in mean lifespan in N2 worms (blue) or eat-2(ad1116) worms (red) treated with RNAi to the indicated genes only during adulthood compared with empty vector. Mean percent change of 1–4 independent experiments is shown. 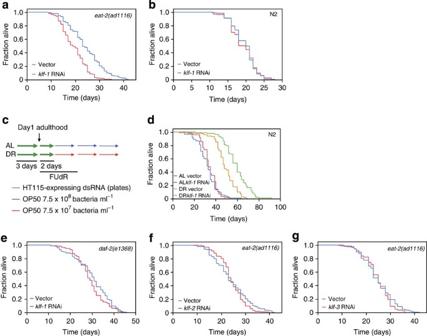* P <0.05, ** P <0.0001 (compared with same strain worms grown on HT115 bacteria harbouring the RNAi plasmid vector; Mantel–Cox log-rank test). Lifespan values are given in Supplementary Table 1 . Figure 2:klf-1is required and specific for the extension of lifespan by dietary restriction. Lifespan curves represent combined data from multiple independent experiments. Lifespan values are given inSupplementary Table 2. (a,b) Lifespan analysis ofeat-2(ad1116)mutant worms (a) or N2 worms (b) fed bacteria expressingklf-1dsRNA only during adulthood or control vector. (c) Schematic representation of liquid culture bacterial dilution experiments with RNAi. (d) Lifespan analysis of N2 worms grown in diet restricted (DR) orad libitum(AL)E. coli(OP50) concentrations in liquid culture from day 3 adulthood after feeding bacteria expressingklf-1dsRNA or control vector on plates. (e) Lifespan analysis ofdaf-2(e1368)mutant animals fedklf-1dsRNA only during adulthood or control vector. RNAi depletion ofklf-2orklf-3during adulthood had no effect ondaf-2(e1368)lifespan (data not shown). (f,g) Lifespan analysis ofeat-2(ad1116)mutant worms fed bacteria expressingklf-2(f),klf-3(g) dsRNA only during adulthood or control vector. Full size image Figure 2: klf-1 is required and specific for the extension of lifespan by dietary restriction. Lifespan curves represent combined data from multiple independent experiments. Lifespan values are given in Supplementary Table 2 . ( a , b ) Lifespan analysis of eat-2(ad1116) mutant worms ( a ) or N2 worms ( b ) fed bacteria expressing klf-1 dsRNA only during adulthood or control vector. ( c ) Schematic representation of liquid culture bacterial dilution experiments with RNAi. ( d ) Lifespan analysis of N2 worms grown in diet restricted (DR) or ad libitum (AL) E. coli (OP50) concentrations in liquid culture from day 3 adulthood after feeding bacteria expressing klf-1 dsRNA or control vector on plates. ( e ) Lifespan analysis of daf-2(e1368) mutant animals fed klf-1 dsRNA only during adulthood or control vector. RNAi depletion of klf-2 or klf-3 during adulthood had no effect on daf-2(e1368) lifespan (data not shown). ( f , g ) Lifespan analysis of eat-2(ad1116) mutant worms fed bacteria expressing klf-2 ( f ), klf-3 ( g ) dsRNA only during adulthood or control vector. Full size image We also tested whether the loss of klf-1 suppressed the extended longevity of animals diet restricted by reduced food intake imposed by bacterial dilution in liquid culture [13] , [14] . Ideally we wanted to use a klf-1 -null allele for this experiment, because RNAi depletion cannot be achieved in liquid culture. However, the only two mutant alleles of klf-1 , tm731 and tm1110, do not appear to be null alleles as both have only short intronic sequence deletions and have a wild-type phenotype [3] ( Supplementary Fig. 2 and Supplementary Table 3 ), and, in consequence, we knocked down expression of klf-1 by RNAi from hatching (L1) to day 3 adults before moving them to liquid cultures of OP50 ( Fig. 2c ). Control N2 animals grown under DR conditions had a lifespan of nearly double that of animals fed ad libitum ( Fig. 2d ). Loss of klf-1 did not affect lifespan of animals fed ad libitum . In contrast, the lifespan of klf-1 -depleted animals undergoing DR was significantly shorter when compared with control animals ( Fig. 2d and Supplementary Table 2 ). As these animals were fed bacteria expressing double-stranded RNA (dsRNA) for only the first 5 days of life, temporary RNAi knockdown of klf-1 in these experiments may explain why we did not observe complete suppression of longevity in animals undergoing DR. Indeed, under identical conditions, we observed a partial suppression of DR lifespan with wwp-1 knockdown, while use of a wwp-1 -null allele gave a much stronger effect ( Supplementary Fig. 3 , Supplementary Table 3 and ref. 13 ). These results indicate that reduction of klf-1 expression early in life is sufficient to reduce the extended longevity of DR animals. To determine whether klf-1 was acting specifically to affect the DR pathway, we examined its effect on other pathways that influence longevity. Reduced IIS, by mutation of the insulin/IGF-1 receptor, daf-2 , increases longevity. RNAi depletion of klf-1 , like wwp-1 , had no effect on the long lifespan of insulin/IGF-1 receptor ( daf-2 ) mutants ( Fig. 2e and Supplementary Table 2 ). In addition, we tested whether klf-1 was required for the long lifespan of animals with reduced mitochondrial electron transport chain activity. We observed suppressive effects on lifespan extension in long-lived isp-1 mitochondrial mutant animals with klf-1 knockdown. However, this was not specific for klf-1 , as RNAi-mediated reduction of klf-2 and klf-3 , the two other KLFs in C. elegans , also gave similar minor lifespan reductions ( Supplementary Fig. 4 and Supplementary Table 3 ). In addition, lifespan modulation directed by klf-1 is specific, as RNAi of klf-2 and klf-3 did not reduce the lifespan of eat-2 mutant animals ( Fig. 2f and g and Supplementary Table 2 ). In sum, klf-1 has a specific and essential role in regulating the response to nutrient intake and longevity. wwp-1 and klf-1 function together to regulate longevity klf-1 is primarily expressed in the intestine of the worm [3] , a site where longevity cues are expressed [15] . We asked if klf-1 functions in this tissue to regulate DR-induced longevity. sid-1 encodes a transmembrane protein required for transporting RNAi silencing signals between cells. Loss of sid-1 does not allow dsRNA to be distributed into peripheral cells [16] . Indeed, when eat-2(ad1116);sid-1(qt9) animals were fed bacteria expressing klf-1 dsRNA, we no longer observed a reduction in lifespan ( Fig. 3a and Supplementary Table 2 ), presumably because the klf- 1 dsRNA could not enter the intestinal cells. Lifespans were then performed with eat-2(ad1116);sid-1(qt9) mutant animals in which sid-1 was restored by tissue-specific expression of sid-1 cDNA. sid-1 was rescued in transgenic lines under the control of the gly-19 intestine-expressing promoter or the myo-3 body wall muscle-expressing promoter. Restoring sid-1 in the intestine and feeding klf-1 dsRNA-producing bacteria to deplete klf-1 selectively in the intestine led to complete suppression of long-lived eat-2 mutant lifespan ( Fig. 3b and Supplementary Table 2 ). In contrast, muscle-specific knockdown of klf-1 had no significant effect on lifespan ( Fig. 3c and Supplementary Table 2 ). WWP-1 is also expressed in the intestine [13] . Like klf-1, knockdown of wwp-1 specifically in the intestine, but not muscle, led to suppression of long-lived eat-2 mutant lifespan ( Fig. 3b and c and Supplementary Table 2 ). Taken together, a major site of action of WWP-1 and KLF-1 to regulate the response to DR appears to be the intestine. Figure 3: The intestine is a major site of action of wwp-1 and klf-1 to regulate the dietary restriction response. ( a ) Lifespan analysis of eat-2(ad1116);sid-1(qt9) mutant worms fed bacteria expressing dsRNA to klf-1 or control vector. ( b , c ) Lifespan analysis of eat-2(ad1116);sid-1(qt9) worms with restored SID-1 expression in the intestines ( b ) or muscle tissues ( c ). Worms were fed bacteria expressing dsRNA to klf-1 , wwp-1 or control vector. Full size image Because loss of klf-1 suppressed longevity, we asked if increased expression of klf-1 was sufficient to increase longevity. We were unsuccessful in generating stable klf-1 transgenic lines by microinjection of a plasmid containing the entire coding sequence of klf-1 and 2 kbp of 5′ upstream sequence from its ATG at low concentrations. Several possibilities could account for our inability to achieve overexpression of klf-1 , including expression levels as well as spatial control of expression. For this reason, we tested whether spatially controlled ectopic expression of klf-1 could influence longevity by generating a transgenic line carrying an intestine-specific construct that expressed klf-1 cDNA fused to a C-terminal tdTomato fluorescent protein. We found that tdTomato expression was very low in this line compared with control lines that express tdTomato alone under the same promoter ( Supplementary Fig. 5a ), suggesting that KLF-1 overexpression may be toxic. Nevertheless, KLF-1 was specifically expressed, as the tdTomato fluorescent signal was reduced on klf-1 dsRNA treatment, but not control vector ( Supplementary Fig. 5b ). We found that this modest level of overexpression of klf-1 in worms extends lifespan by approximately 15%, and this extension was reverted with klf-1 dsRNA treatment ( Fig. 4a and Supplementary Table 2 ). This extension is similar to that we find with wwp-1 overexpression ( Fig. 4d , Supplementary Table 2 and ref. 13 ). The increase in longevity induced by klf-1 expression was suppressed when wwp-1 expression was reduced by RNAi, indicating that the ability of klf-1 to extend lifespan requires wwp-1 ( Fig. 4b and Supplementary Table 2 ). Knockdown of pha-4 , the FoxA transcription factor required for DR-induced longevity [14] , also suppressed the extended lifespan of klf-1 -overexpressing animals ( Fig. 4c and Supplementary Table 2 ) placing klf-1 in the same pathway as pha-4 . Figure 4: wwp-1 and klf-1 function together to regulate diet-restriction-induced longevity. ( a – c ) Lifespan analysis of worms overexpressing KLF-1 in the intestine (KLF-1 o/e) or control worms fed bacteria expressing klf-1 ( a ), wwp-1 ( b ) or pha-4 ( c ) dsRNA from hatching (L1) or control vector. ( d ) Lifespan analysis of WWP-1-overexpressing worms (WWP-1 o/e) or control worms fed bacteria expressing klf-1 dsRNA from hatching (L1) or control vector. Full size image Increased expression of wwp-1 extends the lifespan of N2 worms [13] ( Fig. 4d and Supplementary Table 2 ). Stable transgenic lines that express an N-terminal green fluorescent protein–WWP-1 fusion protein, under the control of the endogenous wwp-1 promoter live longer than control animals [13] . Knockdown of klf-1 suppressed the extended lifespan of wwp-1 -overexpressing animals ( Fig. 4d and Supplementary Table 2 ), indicating that wwp-1 requires klf-1 to extend longevity and that klf-1 functions in the same pathway as wwp-1 to regulate longevity in response to diet. WWP-1 associates with and ubiquitylates KLF-1 The ubiquitin ligase activity of WWP-1 is essential for DR-induced longevity, indicating that WWP-1 functions to ubiquitylate a substrate(s) to mediate its longevity effects [13] . Our genetic analysis of klf-1 suggests that WWP-1 may target KLF-1 for ubiquitylation. Based on these data, we first investigated whether WWP-1 could directly interact with KLF-1. On co-expression of FLAG-tagged KLF-1 and hemagglutinin protein (HA)-tagged WWP-1 in human HEK293T cells, WWP-1 was co-immunoprecipitated with KLF-1 ( Fig. 5a ). To determine if this interaction is direct, we performed pull-down studies using GST–WWP-1 fusion proteins and 35 S-labelled in vitro -translated KLF-1 and found that GST–WWP-1 could pull down KLF-1, whereas GST protein alone did not ( Fig. 5b , left panel). In contrast, the transcription factor PHA-4 did not bind to WWP-1 under the same conditions ( Fig. 5b , right panel). A GST fusion protein containing only the WW domains of WWP-1 (aa 215–412) was sufficient to bind KLF-1, showing that the WW domains of WWP-1 mediate the interaction between KLF-1 and WWP-1 ( Fig. 5c ). These results indicate that WWP-1 can form a complex with KLF-1. 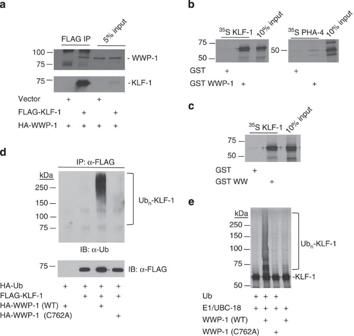Figure 5: WWP-1 associates with and ubiquitylates KLF-1. (a) HA-WWP-1 and FLAG-KLF-1 were expressed in HEK293T cells. Lysates were immunoprecipitated with FLAG antibodies and probed with antibodies against HA (top panel) or FLAG (bottom panel). Molecular size in kilodaltons (kDa) is indicated on the left. (b) GST pull-down assay in which GST–WWP-1 or GST alone bound to glutathione beads was incubated within vitro-translated35S-labelled KLF-1 (left panel) or PHA-4 (right panel). (c) GST pull-down with35S-labelled KLF-1 and a GST fusion protein containing only the WW domains of WWP-1. (d)In vivoubiquitylation of KLF-1 by WWP-1. HEK293T cells were transfected with HA-tagged ubiquitin and FLAG-KLF-1 and/or HA-WWP-1. Denatured lysates were immunoprecipitated with anti-FLAG beads and analysed by immunoblot with an ubiquitin antibody. Similar banding pattern was seen when probed with an anti-HA antibody (data not shown). Bottom panel shows that similar amounts of KLF-1 were immunoprecipitated. (e)In vitroubiquitylation assay using35S-labelled KLF-1 incubated with bacterially expressed recombinant E1, UBC-18 and GST–WWP-1. Recombinant ubiquitin was added to the reaction where indicated. Uncropped images from the autoradiography scans and immunoblots are shown inSupplementary Fig. 9. Figure 5: WWP-1 associates with and ubiquitylates KLF-1. ( a ) HA-WWP-1 and FLAG-KLF-1 were expressed in HEK293T cells. Lysates were immunoprecipitated with FLAG antibodies and probed with antibodies against HA (top panel) or FLAG (bottom panel). Molecular size in kilodaltons (kDa) is indicated on the left. ( b ) GST pull-down assay in which GST–WWP-1 or GST alone bound to glutathione beads was incubated with in vitro -translated 35 S-labelled KLF-1 (left panel) or PHA-4 (right panel). ( c ) GST pull-down with 35 S-labelled KLF-1 and a GST fusion protein containing only the WW domains of WWP-1. ( d ) In vivo ubiquitylation of KLF-1 by WWP-1. HEK293T cells were transfected with HA-tagged ubiquitin and FLAG-KLF-1 and/or HA-WWP-1. Denatured lysates were immunoprecipitated with anti-FLAG beads and analysed by immunoblot with an ubiquitin antibody. Similar banding pattern was seen when probed with an anti-HA antibody (data not shown). Bottom panel shows that similar amounts of KLF-1 were immunoprecipitated. ( e ) In vitro ubiquitylation assay using 35 S-labelled KLF-1 incubated with bacterially expressed recombinant E1, UBC-18 and GST–WWP-1. Recombinant ubiquitin was added to the reaction where indicated. Uncropped images from the autoradiography scans and immunoblots are shown in Supplementary Fig. 9 . Full size image To determine if the interaction between these two proteins results in ubiquitylation of KLF-1 in vivo , we transfected HEK293T cells with HA-tagged ubiquitin, FLAG-KLF-1 and HA-WWP-1. Immunoblot analysis of immunoprecipitated FLAG-KLF-1 from the denatured extracts with an ubiquitin antibody revealed a ladder of bands representing ubiquitylated KLF-1 that was absent when HA-WWP-1 was not expressed or with expression of a catalytically inactive WWP-1 mutant (C762A) ( Fig. 5d ). The ability of WWP-1 to promote ubiquitylation of KLF-1 was confirmed by performing an in vitro ubiquitylation assay using bacterially expressed E1, UBC-18 (E2) and WWP-1 (E3) and 35 S-labelled in vitro -translated KLF-1 substrate. On addition of WWP-1, we observed a ladder of more slowly migrating bands of KLF-1 that was not observed when we used the catalytically inactive WWP-1(C762A) mutant protein ( Fig. 5e ). This modification is ubiquitylation, as its presence was dependent on the addition of recombinant ubiquitin. KLF-1 is preferentially monoubiquitylated by WWP-1 As various types of ubiquitin modification are linked to distinct physiological functions, we investigated the type of ubiquitylation occurring on KLF-1 mediated by WWP-1. Ubiquitin can be covalently conjugated to substrates in several ways. A single ubiquitin can be conjugated to a single site (monoubiquitylation) or multiple sites (multiple monoubiquitylation), or multiple ubiquitins can be linked via one of the seven lysine residues on ubiquitin to form polyubiquitin chains (polyubiquitylation). K48-linkages are abundant, being the predominant signal for proteins destined for degradation by the proteasome. Immunoblot analysis of immunoprecipitated FLAG-KLF-1 from HEK293T cells with an antibody that specifically recognizes K48-linked polyubiquitin chains revealed no difference in the level of ubiquitylated species when KLF-1 was expressed with WWP-1 compared with vector or WWP-1 (C762A) mutant ( Fig. 6a , left panel). We detected a slight increase in KLF-1 high-molecular weight bands with WWP-1 WT expression when the same experiment was probed with an antibody that specifically recognizes polyubiquitylated substrates but not monoubiquitylated substrates ( Fig. 6a , right panel). In contrast, we saw a significantly greater increase of ubiquitylated bands with an antibody that recognizes both polyubiquitylated and monoubiquitylated species ( Fig. 6a , middle panel), indicating that these bands represent KLF-1 conjugated with a ubiquitin monomer at multiple sites. 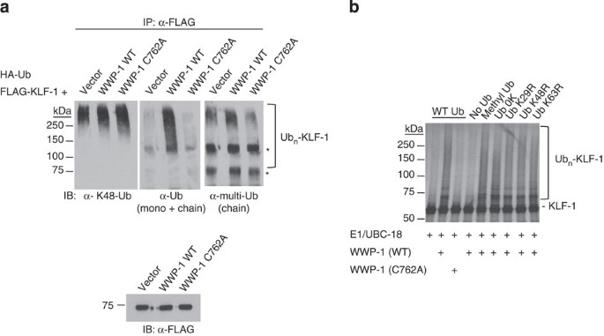Figure 6: KLF-1 is preferentially monoubiquitylated by WWP-1. (a)In vivoubiquitylation assay similar toFig. 5dexcept 0.1 mM Bortezomib was added to the cells. Denatured lysates were immunoprecipitated with anti-FLAG beads and analysed by immunoblot with the indicated ubiquitin antibodies. The asterisks (*) indicate nonspecific bands present in all samples. Bottom panel shows that similar amounts of KLF-1 were immunoprecipitated. (b)In vitroubiquitylation assay using35S-labelled KLF-1 incubated with bacterially expressed recombinant E1, UBC-18 and GST–WWP-1. Recombinant WT ubiquitin or the indicated ubiquitin mutants were added to the reaction where indicated. Uncropped images from the autoradiography scan and immunoblots are shown inSupplementary Fig. 10. Figure 6: KLF-1 is preferentially monoubiquitylated by WWP-1. ( a ) In vivo ubiquitylation assay similar to Fig. 5d except 0.1 mM Bortezomib was added to the cells. Denatured lysates were immunoprecipitated with anti-FLAG beads and analysed by immunoblot with the indicated ubiquitin antibodies. The asterisks (*) indicate nonspecific bands present in all samples. Bottom panel shows that similar amounts of KLF-1 were immunoprecipitated. ( b ) In vitro ubiquitylation assay using 35 S-labelled KLF-1 incubated with bacterially expressed recombinant E1, UBC-18 and GST–WWP-1. Recombinant WT ubiquitin or the indicated ubiquitin mutants were added to the reaction where indicated. Uncropped images from the autoradiography scan and immunoblots are shown in Supplementary Fig. 10 . Full size image To further address whether the observed pattern represented polyubiquitylation or multiple monoubiquitylation, various ubiquitin mutants were analysed in our in vitro assay. The use of methylated ubiquitin, which prevents formation of polyubiquitin chains via its lysine residues, or a recombinant ubiquitin, in which all seven lysine residues of ubiquitin were mutated to arginines (K0), generated a pattern similar to WT ubiquitin. Analysis of single lysine ubiquitin mutants, K29R, K48R and K63R also resulted in a similar banding pattern ( Fig. 6b ). Therefore, it appears that the banding pattern found in our in vitro assay resembles multiple monoubiquitylation of KLF-1 by WWP-1. Taken together, our findings suggest that WWP-1 preferentially catalyses attachment of mono- rather than polyubiquitin moieties to KLF-1. Our study identifies the C. elegans KLF, KLF-1 as a substrate for ubiquitylation by WWP-1. Mammalian orthologues of WWP-1 have been shown to target multiple transcription factors for proteasome-dependent degradation including KLF5 (refs 9 , 10 ), KLF2 (ref. 8 ), Oct-4 (ref. 17 ), Runx2 (ref. 18 ), p63 (ref. 19 ), p73 (ref. 20 ), JunB and cJun [21] . Ubiquitin modifications mediated by mammalian WWP-1 orthologues that do not lead to proteasome-dependent proteolysis have also been found to regulate transcription factor activity. For example, WWP1 increases the transcriptional activity of a p63 isoform (ΔN63) through generation of Lys63-linked polyubiquitin chains [22] . WWP2 monoubiquitylates the homeodomain transcription factor Goosecoid (Gsc), which augments its transcriptional activity [23] . Monoubiquitylation of TIEG1/KLF10 by Itch has been shown to directly regulate KLF10 transcriptional activity, while K27-linked ubiquitylation by the same E3 modulates its cellular localization (described above) [11] , [12] . In addition, Itch suppresses the transactivation activity of p45/NF-E2 by the addition of a K63-linked chain causing it to be retained in the cytoplasm [24] , while monoubiquitylation of p53 by WWP1 negatively regulates its transcriptional activity by shuttling it to the cytoplasm [25] . Our genetic data indicate that klf-1 , like wwp-1, is a positive regulator of lifespan suggesting that KLF-1 activity is enhanced on DR. Our data support a model in which ubiquitylation of KLF-1 by WWP-1 regulates the DR-longevity response. While we were able to demonstrate WWP-1-dependent ubiquitylation of KLF-1 both in vitro and in cellulo , we were not able to detect ubiquitylation of KLF-1 in the worm. This may be a detection problem due to the low expression of tagged KLF-1 in our transgenic animals. However, our results using these two systems indicate that WWP-1 mediates multiple monoubiquitylation of KLF-1. As monoubiquitylation does not signal proteasome-mediated degradation, KLF-1 modification by WWP-1 should not affect its stability. Indeed, we did not observe discernable differences in tdTomato fluorescence when wwp-1 was knocked down in worms that express KLF-1-tdTomato fusion protein in the intestine ( Supplementary Fig. 6 ). It is unclear how WWP-1-mediated ubiquitylation of KLF-1 would affect its function in the intestine. KLF-1 ubiquitylation might cause a change in subcellular localization, so that KLF-1 is not available for proteasome-dependent degradation. However, we did not observe an obvious change in the cytoplasmic and nuclear localization of KLF-1 when expressed with WT WWP-1 or the C762A mutant, as determined by immunofluorescence in HEK293T cells ( Supplementary Fig. 7 ). KLF-1 ubiquitylation by WWP-1 might alter the ability of KLF-1 to regulate gene transcription, for instance, by regulating KLF-1 binding to transcriptional regulators or specific gene promoters [26] . At this time, target genes regulated by KLF-1 in the worm have not been identified. It is unlikely that KLF-1 mediates transcription of stress response genes, as knockdown of klf-1 did not confer sensitivity to various stresses, including mild heat stress, oxidative stress and ultraviolet ( Supplementary Fig. 8 and Supplementary Table 3 ). Previous studies have reported that loss of klf-1 results in increased fat storage in the intestine and cell death in the germline [3] . Recent research has shown direct links between lipid metabolism, germline control and longevity [27] , [28] . Defects in fat metabolism and/or germline maintenance may contribute to the suppression of DR-induced longevity with loss of klf-1 . Indeed, worms undergoing DR have reduced intestinal fat stores, and loss of klf-1 causes an increase of fat storage in the intestine [3] . It is believed that most of the life-extending benefits of DR are a consequence of its ability to reduce fat stores. In mice, long-term DR results in a shifted transcriptional phenotype reflecting energy metabolism activation in adipose tissue [29] . It is intriguing to speculate that klf-1 may regulate lipid status in the worm, which in turn affects aging, especially given that the C. elegans intestine is the major organ involved in lipid metabolism and is an important target organ in mediating lifespan extension [30] . Indeed, several mammalian KLF family members have been identified to be key players in the transcription of genes that control adipogenesis, lipogenesis and obesity [2] . Possibly, klf-1 exerts its role in the intestine via transcriptional regulation of genes modulating the activity of signalling pathways that control fat metabolism. Genes directly involved in lipid metabolism have been mapped to several signalling pathways that affect longevity including DR [31] . However, the exact role of lipids in modulation of aging remains unclear. Gene expression studies of worms with intestine-specific knockdown of WWP-1 and/or KLF-1 could help clarify the role of WWP-1 and KLF-1 in the DR pathway. Perhaps C. elegans klf-1 , like pha-4 , feeds into the target of rapamycin pathway to regulate longevity [32] . Indeed, we do find a genetic interaction between pha-4 and klf-1 in regulating DR-induced longevity. There are numerous examples of Forkhead transcription factors regulating expression of KLFs and vice versa. For example, Drosophila forkhead binds to the Krüppel gene promoter and upregulates Krüppel gene expression [33] and mammalian FOXO1 regulates KLF2, KLF4 and KLF6 expression [34] , [35] , [36] . In addition, KLF4 has been shown to negatively regulate expression of FOXM1 (ref. 37 ) and ubiquitylated KLF10 upregulates FOXP3 expression [11] . Further dissection of the transcription network involving KLF-1 and PHA-4 would be critical in advancing our understanding of how DR enhances longevity. C. elegans strains and methods Nematodes were handled using standard methods [38] . WWP-1-overexpressing transgenic animals (P wwp-1 ::green fluorescent protein::WWP-1) and the control line (P wwp-1 ::green fluorescent protein) have been previously described [13] . Generation of transgenic lines Extrachromosomal arrays carrying transgenic strains were generated using standard microinjection methods [39] . For generation of N2 animals overexpressing klf-1 , P gly-19:: KLF-1::tdTomato plasmid DNA was injected with the pRF4 ( rol-6 ) construct. N2 animals injected with pRF4 were used as a control. For generation of eat-2(ad1116);sid-1(qt9) mutant animals with restored tissue-specific expression of SID-1, P gly-19 ::SID-1 plasmid DNA was injected with P gly-19 ::tdTomato plasmid DNA (for expression in intestinal tissue) or P myo-3 ::SID-1 plasmid DNA was injected with P myo-3 ::tdTomato (for expression in muscle tissue). Individual transgenic F 1 progeny were selected on the basis of roller phenotype or tdTomato expression. Transgenic F 2 animals were isolated to establish independent lines. Lifespan analysis For lifespan analyses, synchronized populations of eggs were hatched and allowed to develop to the L4 stage. Once in the L4 stage, worms were transferred to new plates. The first day of adulthood is day 1 in survival curves. Worms were transferred to new plates every 24 h during the first six days of adulthood to eliminate confounding progeny. Animals were scored as alive, dead or censored every 2–3 days. Worms were scored as dead if they did not respond to repeated prods with a platinum pick. Animals that crawled off the plate, exploded or bagged were censored at the time of event. All lifespans were performed at 20 °C unless noted. Lifespan curves represent combined data from multiple independent experiments. eat-2(ad1116) ;CF512 larvae were plated at the restrictive temperature (25 °C) at day 1 of adulthood and then moved to and maintained at 20 °C for the remainder of the lifespan. For bacterial dilution liquid culture lifespans, synchronized populations of eggs were hatched and grown at 20 °C on nematode growth (NG) agar plates containing OP50 Escherichia coli until the L4 larval stage when they were transferred to plates of OP50 containing 100 μg ml −1 FUdR (to block worm reproduction). At day 1 of adulthood, worms were transferred into liquid culture containing OP50 bacteria at a concentration of either 7.5 × 10 7 cells ml −1 (DR) or 7.5 × 10 8 cells ml −1 (AL). Liquid cultures contained FUdR at 100 μg ml −1 for the first 4 days. Animals were transferred to new liquid cultures every 3–4 days and were scored as alive, dead or censored at the time of transfer. For bacterial dilution liquid cultures with RNAi knockdown, synchronized populations of eggs were hatched and grown on NG-carb agar plates containing bacteria expressing klf-1 dsRNA, wwp-1 dsRNA or vector control to D1 adults when they were transferred to plates containing dsRNA-expressing bacteria and 100 μg ml −1 FUdR. At day 3 of adulthood, worms were transferred to liquid cultures containing OP50 bacteria at either DR or AL concentrations. Statistical analysis JMP8 software was used to determine means and percentiles. P values were calculated using the log-rank (Mantel–Cox method). P values were calculated for individual experiments, each consisting of control and experimental animals examined at the same time. P values were also calculated for combined data from multiple identical experiments. RNAi treatment RNAi-treated strains were fed E. coli (HT115) containing an empty vector or E. coli expressing dsRNA against the gene of interest. Unless indicated, worms were fed bacteria expressing dsRNA from hatching (L1). The wwp-1, pha-4, klf-2, ama-1, let-23, sek-1, mkk-4, rnt-1, ceh-6, lin-12 and hgrs-1 RNAi clones were from Julie Ahringer’s RNAi library [40] . RNAi clones against klf-1, klf-3 and jun-1 were from Marc Vidal’s RNAi library [41] . Pumping rates Pumping rates were determined by counting pumps of the terminal pharyngeal bulb for 1 min intervals. For each condition, worms were treated with bacteria expressing dsRNA since hatching. The pumping rates of 10 D1 adult worms per condition were measured and averaged. Stress assays For ultraviolet irradiation assays, worms were hatched and grown on specific RNAi-treated plates. At the L4 stage of development 100 μg ml −1 FUdR was added to the plates. D1 adults were transferred to plates without food and exposed to 1,200 J m −2 ultraviolet radiation using a Stratalinker UV Crosslinker (Stratagene). Worms were transferred back to fresh plates seeded with appropriate RNAi treatments and scored daily for viability. For paraquat (methyl viologen, Sigma) assays, worms were submerged in 50 μl of 0.4 M paraquat dissolved in S-basal buffer at day 5 of adulthood, after reproduction had ceased. Death was determined on an hourly basis by the lack of movement after prodding with a platinum wire. All assays were performed at 20 °C. Plasmids and cell transfection To generate N-terminally-tagged HA-WWP-1, wwp-1 (WT and C762A mutant) were subcloned into the pcDNA3 mammalian expression plasmid that had HA sequence inserted into the polylinker region. klf-1 cDNA cloned into pDONR201 was obtained from Open Biosystems. klf-1 was subcloned into the pCMV-3Tag-1 vector (Agilent Technologies) to generate N-terminally-tagged Flag 3 -KLF-1 for mammalian expression. The ubiquitin construct used, which expresses eight tandem copies of HA-tagged ubiquitin under the control of the CMV promoter, has been previously described [42] . HEK293T cells were transfected with expression plasmids using polyethylenimine (Sigma) and collected 30 h later. Where indicated, 1 μM bortezomib (Selleck Chemicals) was added to cells 24 h after transfection. Samples were harvested 6 h after bortezomib treatment. Immunoprecipitation and immunoblot assays For immunoprecipitation assays, cell pellets were resuspended in 1% NP40 lysis buffer (50 mM Tris–HCl (pH 8.0), 150 mM NaCl, 1% NP40; the following was added to the buffer before lysis: 1 mM dithiothreitol, 0.1 mM Na 3 VO 4 , 0.1 mM phenylmethylsulphonyl fluoride, 1 μg ml −1 aprotinin). FLAG-KLF-1 was immunoprecipitated using anti-FLAG M2 affinity gel (Sigma). Immunoprecipitates were washed four times with lysis buffer and subjected to SDS–polyacrylamide gel electrophoresis. Gels were transferred to polyvinylidene difluoride membranes and probed with a monoclonal HA epitope tag antibody (ascites fluid from 12CA5 hybridoma cells) at a dilution of 1/10,000 to detect HA-WWP-1 and a monoclonal FLAG M2 epitope tag antibody (Sigma) at a dilution of 1/1,000 to detect FLAG-KLF-1. Immunofluorescence assays For immunofluorescence assays, HEK293T cells were plated on glass coverslips and transfected with the indicated plasmids. Cells were then fixed with 4% paraformaldehyde and stained with a monoclonal anti-FLAG antibody (M2) (Sigma) at a dilution of 1/1,000 μl to detect KLF-1 expression, followed by incubation with a mouse secondary antibody (IgG) conjugated to Alexa Fluor 488 (Molecular Probes) at a dilution of 1/500. Cells were counterstained with Hoechst to identify all nuclei before mounting on slides. Microscopy For fluorescence microscopy of transgenic worms, worms were anesthetized with 50 mM sodium azide on NG agar plates and were analysed using a Leica S6E dissecting microsope. Immunostained 293T cells were analysed using a Leica 6000B digital microscope. Images were acquired using Leica FW4000 and AF6000 software. In vivo ubiquitylation assay Transfected cells were washed two times with phosphate-buffered saline containing 2 mM N -ethyl maleimide (to block the activity of isopeptidases and deubiquitylating enzymes). Cells were immediately lysed on the plate with preheated (95 °C) 2% SDS lysis buffer (50 mM Tris–HCl (pH 7.4), 150 mM NaCl, 2% SDS; the following was added to the buffer immediately before lysis: 1 mM dithiothreitol, 0.1 mM Na 3 VO 4 , 0.1 mM phenylmethylsulphonyl fluoride, 1 μg ml −1 aprotinin and 4 mM N -ethyl maleimide). Lysates were boiled for 10 min. Denatured samples were then diluted in 1% Triton X-100 lysis buffer (50 mM Tris–HCl (pH 7.4), 150 mM NaCl, 1% Triton X-100; the following was added to the buffer immediately before lysis: 1 mM dithiothreitol, 0.1 mM Na 3 VO 4 , 0.1 mM phenylmethylsulphonyl fluoride, 1 μg ml −1 aprotinin and 2 mM N -ethyl maleimide) so that the final volume of SDS was reduced to 0.1%. Cells were left on ice for 30 min and insoluble material was removed by centrifugation. Anti-FLAG M2 affinity gel (Sigma) was added to the lysates and incubated overnight at 4 °C. Immunoprecipitates were washed four times with 1% Triton X-100 lysis buffer and subjected to SDS–polyacrylamide gel electrophoresis. Gels were transferred to polyvinylidene difluoride membranes and probed with the mouse monoclonal multi-ubiquitin FK1 antibody (MBL), which recognizes K6-, K11-, K27-, K33-, K29-, K48- and K63-linked ubiquitin chains but not monoubiquitin linkages. After stripping, the membrane was then probed with the mouse monoclonal P4D1 ubiquitin antibody (Santa Cruz) to detect total ubiquitin conjugates (polyubiquitin and monoubiquitin linkages). The membrane was then stripped again and probed with the rabbit polyclonal K48-specific ubiquitin antibody Apu2 (Millipore). The FK1, P4D1 and Apu2 antibodies were used at a dilution of 1/1,000. Similar results were seen in an identical independent experiment where the membrane was first probed with the Apu2 antibody (data not shown). Recombinant proteins and GST pull-down experiments His-E1, GST–WWP-1 (WT and C762A mutant) and UBC-18 recombinant proteins have been previously described [13] . The WW domain-containing region of WWP-1 (Amino acids 215–412) was cloned by PCR and subcloned into the pGEX6P1 bacterial expression vector to generate GST-WW. GST purifications were performed according to the manufacturer’s instructions. klf-1 and pha-4 cDNAs were subcloned into the pCRII vector (Invitrogen) and used in the TnT Coupled Transcription/Translation Systems (Promega) to produce 35 S-methionine-labelled protein. For pull-down experiments, 5 or 10 μl of 35 S-labelled lysates were incubated with 3.3 μg of GST or GST fusion protein bound to glutathione beads in binding buffer (50 mM Tris–HCl (pH 8.0), 200 mM NaCl, 1 mM EDTA, 1% NP40, 10 mM MgCl 2 and 1 mM dithiothreitol) for 2 h at 4 °C. Beads were washed four times with binding buffer and analysed by SDS–polyacrylamide gel electrophoresis. 35 S-labelled proteins were identified by autoradiography. In vitro ubiquitylation assay The ubiquitylation reaction mix contained 20 μg WT ubiquitin, ubiquitin mutants or methyl ubiquitin (Boston Biochem), 1 μM ubiquitin aldehyde, 0.5 μg His-E1, 0.2 μg UBC-18, 0.25 μg GST–WWP-1 (WT or C762A mutant) and 1 μl in vitro -translated 35 S-labelled KLF-1 in 10 μl reaction buffer (50 mM Tris–HCl, pH 7.5, 5 mM MgCl 2 , 1 mM dithiothreitol and 5 mM ATP). Following incubation at 30 °C for 90 min, ubiquitylation reactions were stopped with sample buffer and run on protein gels under denaturing conditions. Ubiquitylated KLF-1 forms were identified by autoradiography. How to cite this article: Carrano, A. C. et al. A Krüppel-like factor downstream of the E3 ligase WWP-1 mediates dietary-restriction-induced longevity in Caenorhabditis elegans . Nat. Commun. 5:3772 doi: 10.1038/ncomms4772 (2014).